Robust carbon dioxide reduction on molybdenum disulphide edges Electrochemical reduction of carbon dioxide has been recognized as an efficient way to convert carbon dioxide to energy-rich products. Noble metals (for example, gold and silver) have been demonstrated to reduce carbon dioxide at moderate rates and low overpotentials. Nevertheless, the development of inexpensive systems with an efficient carbon dioxide reduction capability remains a challenge. Here we identify molybdenum disulphide as a promising cost-effective substitute for noble metal catalysts. We uncover that molybdenum disulphide shows superior carbon dioxide reduction performance compared with the noble metals with a high current density and low overpotential (54 mV) in an ionic liquid. Scanning transmission electron microscopy analysis and first principle modelling reveal that the molybdenum-terminated edges of molybdenum disulphide are mainly responsible for its catalytic performance due to their metallic character and a high d -electron density. This is further experimentally supported by the carbon dioxide reduction performance of vertically aligned molybdenum disulphide. During the last few decades, the amount of carbon dioxide (CO 2 ) present in the environment has reached the highest level (396.80 p.p.m.) of the last 20 million years [1] , causing radical and largely unpredictable changes in the environment [2] , [3] , [4] . Recent efforts have revealed that CO 2 can be converted by electrochemical reduction processes using renewable energy sources into energy-rich modules, offering an efficient path for both CO 2 remediation and an alternative energy source [5] , [6] , [7] , [8] , [9] . However, the CO 2 reduction by electrochemical processes faces various fundamental and practical challenges mainly due to high-cost and unsatisfactory conversion performance of existing catalytic systems [5] . Numerous physical and chemical approaches have been employed to improve the performance of existing CO 2 reduction systems [10] , [11] , [12] , [13] , [14] without achieving a major breakthrough. Recently, molybdenum disulphide (MoS 2 ) and related layered materials have attracted a significant attention due to their low price and prominent catalytic features. MoS 2 became widely used as an efficient catalyst for hydrodesulphurization [15] , [16] , oxygen reduction reactions [17] and hydrogen evolution reaction (HER) [16] , [17] . Moreover, it was demonstrated that MoS 2 has a noteworthy performance for water splitting, approaching that of Pt-group metals [17] , [18] , [19] . In this study, we report that layer-stacked bulk MoS 2 with molybdenum (Mo)-terminated edges exhibits the highest CO 2 reduction performance reported to date, to the best of our knowledge. This performance is demonstrated in a diluted solution of 1-ethyl-3-methylimidazolium tetrafluoroborate (EMIM-BF 4 ) ionic liquid that is, 4 mol% EMIM-BF 4 and 96 mol% water. EMIM-BF 4 is deliberately selected due to its’ particular catalytic features, which make the system more selective for carbon monoxide (CO) formation than hydrogen (H 2 ) production [7] , [8] , [9] . In the same diluted electrolyte, commonly used silver nanoparticles (Ag NPs) exhibit moderate performance, whereas a bulk silver (Ag) catalyst is unable to reduce CO 2 . The high catalytic activity of bulk MoS 2 is attributed to the Mo-terminated edges, where the Mo atoms possess approximately one order of magnitude higher ( d orbital) electronic density than Ag atoms at the surface of an Ag film, as shown by our first principle calculations. The lower work function (3.9 eV) also promotes the advanced performance of the MoS 2 catalyst [20] . The performance of the MoS 2 catalyst is further improved by designing an atomic edge-terminated surface via synthesizing vertically aligned MoS 2 . 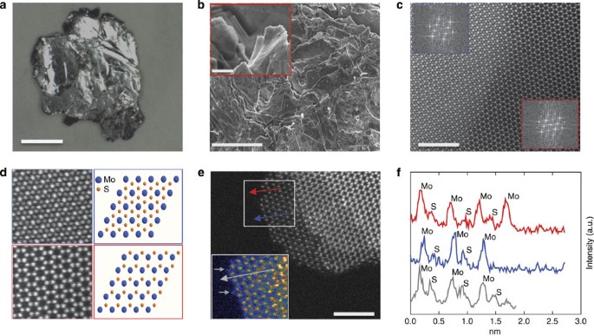Figure 1:Structural and elemental analysis of MoS2. (a) Optical image of bulk MoS2used as catalyst (scale bar, 2 mm), (b) Scanning electron microscopy images of the MoS2displaying the stacked-layered structure and sharp edges of the MoS2flakes. Scale bars are 50 and 5 μm (for inset), respectively, and (c) high-angle annular dark-field (HAADF) images (scale bar, 5 nm) showing both the 1T (blue) and 2H (red) phases of MoS2, along with their respective Fast Fourier Transforms (FFTs) (inset). (d) Higher magnification HAADF images show clearly distinct atomic configuration corresponding to the 1T (top) and 2H (bottom) type of MoS2. The related schematic atomic models have also been shown on the right side. (e) Raw greyscale HAADF and false-color low-angle annular dark-field (LAADF) image (inset) of MoS2edges (scale bar, 5 nm) and (f) the line scans (red and blue towards edges) identifying Mo atoms to be the terminating atoms in the general case. In limited instances, an additional light atom (grey line scan) occupying what should be a Mo-position, most probably a carbon atom, from the STEM substrate. Characterization Figure 1a and b shows optical and scanning electron microscopy images, respectively, of the layered structure [21] , [22] of our bulk MoS 2 sample ( Supplementary Fig. 1 ). Such layered assemblies offer a large number of edges (inset of Fig. 1b ), which are believed to be highly electrocatalytically active sites in electrochemical reactions [17] , [23] . To further detail the atomic arrangement, scanning transmission electron microscopy (STEM) analysis was performed on several mechanically exfoliated, mono- and multi-layer-thick sheets of MoS 2 flakes. Since the STEM high-angle annular dark-field (HAADF) image intensity relies on the atomic number ( Z ), it delivers direct information about the arrangement of Mo and S atoms in the MoS 2 film. The results of the STEM structural ( Fig. 1c ) and Fast Fourier transform analyses ( Supplementary Fig. 2 ) show that the MoS 2 layers are made of two clearly distinct structural domains consisting of 1T (octahedral) and 2H (triangular prismatic). The magnified images (atomic resolution) of selected regions confirm the coexistence of both 1T and 2H atomic arrangements ( Fig. 1d ). Figure 1: Structural and elemental analysis of MoS 2 . ( a ) Optical image of bulk MoS 2 used as catalyst (scale bar, 2 mm), ( b ) Scanning electron microscopy images of the MoS 2 displaying the stacked-layered structure and sharp edges of the MoS 2 flakes. Scale bars are 50 and 5 μm (for inset), respectively, and ( c ) high-angle annular dark-field (HAADF) images (scale bar, 5 nm) showing both the 1T (blue) and 2H (red) phases of MoS 2 , along with their respective Fast Fourier Transforms (FFTs) (inset). ( d ) Higher magnification HAADF images show clearly distinct atomic configuration corresponding to the 1T (top) and 2H (bottom) type of MoS 2 . The related schematic atomic models have also been shown on the right side. ( e ) Raw greyscale HAADF and false-color low-angle annular dark-field (LAADF) image (inset) of MoS 2 edges (scale bar, 5 nm) and ( f ) the line scans (red and blue towards edges) identifying Mo atoms to be the terminating atoms in the general case. In limited instances, an additional light atom (grey line scan) occupying what should be a Mo-position, most probably a carbon atom, from the STEM substrate. Full size image Identification of the atoms on the MoS 2 edges is also crucially important, as the Mo and S atoms possess entirely different electronic structures. Figure 1e shows the edge of a MoS 2 flake imaged in HAADF and low-angle annular dark-field (LAADF) (inset) mode. The line intensity profiles (plotted towards vacuum) suggest that the edges of the MoS 2 flakes are Mo terminated ( Fig. 1f ). This finding is in agreement with the earlier work by Zhou et. al. [24] who report that the Mo-terminated edges have the lowest formation energy in free-standing single-layer MoS 2 . In rare instances, a substitutional defect (atom) appears at the MoS 2 edge. Based on the LAADF image (inset of Fig. 1e ) and the line intensity profile (grey line), it is clear that this is a lighter atom (compared with S), most likely a carbon atom (from the underlying holey carbon STEM grid). Hence, the STEM analysis undoubtedly validates the presence of Mo atoms on the edges of MoS 2 flakes. Catalytic evaluation The CO 2 reduction ability of bulk MoS 2 covered by flakes with exposed Mo-terminated edges was first examined by performing cyclic voltammetry (CV). The applied voltage was swept between +1.0 and −0.764 V versus reversible hydrogen electrode (RHE; in the present study, all potentials are reported with respect to RHE) with a 15 mV s −1 scan rate. The experiments were conducted in a two-compartment three-electrode electrochemical cell ( Supplementary Fig. 3 ) using argon (Ar) or CO 2 -saturated 96 mol% water—4 mol% EMIM-BF 4 solution (pH~4) as an electrolyte. 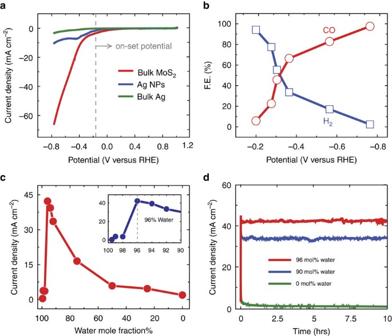Figure 2: CO2reduction performance of the bulk MoS2catalyst in the EMIM-BF4solution. (a) Cyclic voltammetric (CV) curves for bulk MoS2, Ag nanoparticles (Ag NPs) and bulk Ag in CO2environment. The experiments were performed in 96 mol% water and 4 mol% EMIM-BF4solution by sweeping applied potential from +1 V to −0.764 V versus RHE. The vertical grey line indicates the low overpotential (~54 mV) for CO2reduction at bulk MoS2. (b) CO and H2Faradaic efficiency (FE) at different applied potentials. (c) The current density of CO2reduction (measured by Chrono-Amperometry) at 0.764 V versus RHE as a function of water mole fraction in EMIM-BF4electrolyte. The maximum current density was recorded in 96 mol% water - 4 mol% EMIM-BF4electrolyte (inset). The pH value of the solutions was also monitored (Supplementary Table 1). (d) Chrono-Amperometry results of MoS2catalyst in different solutions (96, 90 and 0 mol% water) showing negligible loss in current density even after 10 h. Figure 2a represents the CV curve for the CO 2 reduction. It should be noted that the CO 2 reduction equilibrium potential is −0.11 V versus RHE in the protic media [7] , [10] . We observed that CO 2 reduction reaction initiates at −0.164 V confirmed by measuring CO as a product by gas chromatography (GC) system (CO Faradaic efficiency FE=~3%). This suggests a very low overpotential (54 mV) for CO formation in our system. At −0.2 V (90 mV overpotential), approximately 7% CO formation FE was measured ( Fig. 2b ). MoS 2 also exhibits a significantly high CO 2 reduction current density (65 mA cm −2 at −0.764 V), where CO 2 is selectively converted to CO (FE~98%). However, at the same potential (−0.764 V), the bulk Ag catalyst shows a considerably lower current density (3 mA cm −2 ) ( Fig. 2a ) but for the H 2 formation ( Supplementary Fig. 4a ). Ag NPs (average diameter of 40 nm) show only a current density of 10 mA cm −2 with 65% selectivity for the CO formation under the same experimental conditions ( Fig. 2a and Supplementary Fig. 4b ). In addition, the CO 2 reduction current density for MoS 2 is also significantly higher than the maximum current density (~8.0 mA cm −2 ) achieved when Ag NPs were used in the dynamic electrochemical flow cell using a similar electrolyte solution [13] . For all the cases, the current densities were normalized against the geometrical surface area [9] , [10] , [16] , [17] , [25] , [26] . Surprisingly, the MoS 2 catalyst also shows a high current density (50 mA cm −2 ) in an Ar-saturated electrolyte, where only H 2 was detected as the major product ( Supplementary Note 1 and Supplementary Fig. 5 ). These results are discussed further in supporting information. Figure 2: CO 2 reduction performance of the bulk MoS 2 catalyst in the EMIM-BF 4 solution. ( a ) Cyclic voltammetric (CV) curves for bulk MoS 2 , Ag nanoparticles (Ag NPs) and bulk Ag in CO 2 environment. The experiments were performed in 96 mol% water and 4 mol% EMIM-BF 4 solution by sweeping applied potential from +1 V to −0.764 V versus RHE. The vertical grey line indicates the low overpotential (~54 mV) for CO 2 reduction at bulk MoS 2 . ( b ) CO and H 2 Faradaic efficiency (FE) at different applied potentials. ( c ) The current density of CO 2 reduction (measured by Chrono-Amperometry) at 0.764 V versus RHE as a function of water mole fraction in EMIM-BF 4 electrolyte. The maximum current density was recorded in 96 mol% water - 4 mol% EMIM-BF 4 electrolyte (inset). The pH value of the solutions was also monitored ( Supplementary Table 1 ). ( d ) Chrono-Amperometry results of MoS 2 catalyst in different solutions (96, 90 and 0 mol% water) showing negligible loss in current density even after 10 h. Full size image Figure 2b shows the measured FE of the CO and H 2 formation for a wide range of applied potentials between −0.2 and −0.764 V. Interestingly, depending on the applied potential, MoS 2 effectively operates as a catalyst for both CO 2 reduction and HER. CO 2 is converted at MoS 2 into a tunable mixture of H 2 and CO (syngas), ranging in each component from 0 to ~100%. The variation in FE of CO and H 2 as a function of the applied potential originates from the differences in the CO 2 and HER reduction mechanisms. In principle, the favourable thermodynamic potential for the H 2 evolution is lower than CO 2 reduction. As the applied potential exceeds the onset potential of the CO 2 reduction (−0.164 V), this reaction is activated. Essentially, two H + are consumed for a CO formation as a result of one CO 2 molecule reduction [10] , [13] , [27] , [28] , [29] . Thus, a fraction of both the existing H + (from the electrolyte) and the electrons (on the catalyst surface) are consumed in CO 2 reduction reactions instead of HER reactions. In addition, the EMIM–CO 2 complex works as an inhibitor for the H 2 formation in HER [7] . Here, it is useful to compare the MoS 2 catalyst performance with the existing results for noble metal catalysts ( Fig. 3 and Supplementary Fig. 6 ). It should be noted that current density represents the CO formation rate, whereas FE shows the amount of current density consumed to produce CO during the CO 2 reduction reaction. Thus, we compared the catalysts’ overall performance by multiplying these two parameters at different overpotentials. Interestingly, we noticed that bulk MoS 2 exhibits the highest performance at all overpotentials. At low overpotentials (0.1 V), bulk MoS 2 shows almost 25 times higher CO 2 reduction performance compared with the Au NPs [10] and ~1.3 times higher than the Ag NPs. At higher overpotentials (0.4 V), bulk MoS 2 exhibits approximately one order of magnitude higher performance than Ag NPs and more than two times higher than recently reported nanoporous Ag [14] . At this overpotential, the Au NPs compete with bulk MoS 2 . It should be noted that MoS 2 produce H 2 as a by-product which allows obtaining directly synthetic gas, whereas Au NPs produces formic acid (HCOO − ) as a by-product in the examined conditions [10] . As mentioned previously, bulk Ag is unable to reduce CO 2 in the examined experimental conditions. Moreover, the Cu performance [11] remains below that of Ag NPs, Au NPs and bulk MoS 2 . These results clearly indicate that MoS 2 exhibits the highest CO 2 reduction performance reported so far. 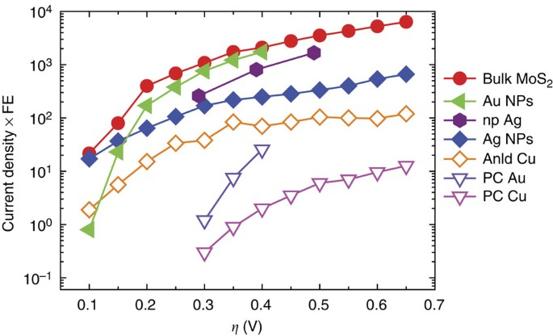Figure 3: Overview of different catalysts’ performance at different overpotentials. Bulk MoS2, Ag nanoparticles (Ag NPs) and bulk Ag results were taken from the present study where electrochemical experiments were performed in similar conditions. Oxidized Au nanoparticles (Au NPs) and polycrystalline Au (PC Au) data were carefully extracted from the reference10. Annealed copper (Anld Cu) and polycrystalline Cu (PC Cu) data were taken from reference11. Nanoporous Ag (np Ag) data were extracted from reference14. CO2reduction performance curve of bulk Ag is not shown as its performance is almost zero in experimental conditions discussed in the text. The extended results are provided in the supporting file. Figure 3: Overview of different catalysts’ performance at different overpotentials. Bulk MoS 2 , Ag nanoparticles (Ag NPs) and bulk Ag results were taken from the present study where electrochemical experiments were performed in similar conditions. Oxidized Au nanoparticles (Au NPs) and polycrystalline Au (PC Au) data were carefully extracted from the reference [10] . Annealed copper (Anld Cu) and polycrystalline Cu (PC Cu) data were taken from reference [11] . Nanoporous Ag (np Ag) data were extracted from reference [14] . CO 2 reduction performance curve of bulk Ag is not shown as its performance is almost zero in experimental conditions discussed in the text. The extended results are provided in the supporting file. Full size image Next, we investigated how the water mole fraction affects the catalytic activity of the MoS 2 catalyst for the CO 2 reduction ( Fig. 2c ). We observe that the CO 2 reduction current density largely grows above 90 mol% water solution densities (inset Fig. 2c ) and reaches a maximum in the 96 mol% water solution. The addition of water molecules can tailor the pH value (that is, H + concentration) of the electrolyte [13] , [30] , [31] ( Supplementary Table 1 ) and consequently affect the electrochemical reduction reaction rate. The pH of the electrolyte fluctuates due to the hydrolysis of BF 4 − , which produces anions (for example, (BF 3 OH) − ) and HF [13] , [30] , [31] . It should be noted that the overall CO 2 -to-CO conversion reaction requires both electrons and protons [13] . Our density functional theory (DFT) calculations show significantly higher density (more than one order of magnitude) of d electrons on Mo-edge atoms compared with Ag (for details, see DFT section), suggesting that the concentration of protons (H + ) is the rate-determining part of the CO 2 reduction reaction. Thus, the attained maximum rate of the reduction process is attributed to: (i) the high concentration of H + (pH~4) in the reaction media and (ii) the low viscosity of the solution. It is clear that the low viscosity allows for a high diffusion rate of the reactants (EMIM–CO 2 − and H + ) towards the catalyst’s active edge sites [27] , [32] , [33] , [34] . A similar trend was observed for Ag NPs catalysts in a dynamic electrochemical flow cell when the maximum current density (~8 mA cm −2 ) was obtained in a 90 mol% water electrolyte [13] . Additionally, a catalyst’s stability is a major issue to be addressed. Thus, we examined the stability of the catalyst for a prolonged period (10 h) in 96, 90 and 0 mol% water solutions. As seen in Fig. 2d , the steady-state current densities remain stable for the studied time (10 h), providing evidence of the long-term stability and efficiency of the MoS 2 catalyst. To elucidate the origin of the high CO 2 reduction rate on the MoS 2 catalyst, we calculated its projected density of states (PDOS) per different Mo and S atoms [20] , [35] , [36] , using DFT methods (for computational details, see method section). The density of states at the Fermi energy level ( E f ) roughly determines the availability of electrons for a given reaction [35] . We found that the electronic structure of MoS 2 ribbons ( Supplementary Note 2 ) is near E f formed by edge bands of only one-spin polarization, originating from the Mo and S atoms exposed at both MoS 2 edges. In the vicinity of E f, the spin-polarized PDOS for these Mo atoms is approximately twice larger than that of the bulk Mo atoms ( Fig. 4a ). Since the bulk Mo atoms, sandwiched between two S layers, are not directly exposed to the electrolyte, the MoS 2 catalytic activity should be primarily related to the edge states formed by Mo-edge atoms ( Supplementary Fig. 7 ). The S atoms possess less reactive p orbitals ( Supplementary Fig. 8 ), and they are not present at the catalytically active edge sites (confirmed by STEM). 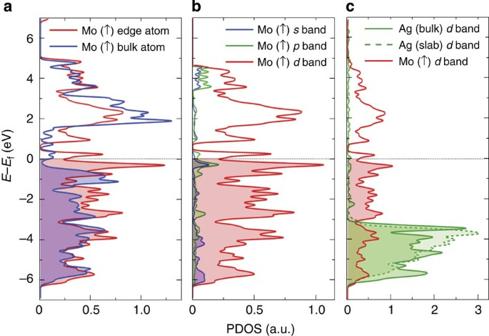Figure 4: DFT calculations of electron density. PDOSs for spin-up channel of: (a) the Mo atom at the edge and Mo atom within the lattice; (b)s,p, anddorbital of Mo-edge atom. (c) PDOS ofdband of Mo-edge atom, Ag atom from bulk and Ag-slab of 8.32-Å thickness. Electron density on Mo-edge atom is significantly (~11 times) higher than the electron density on Ag atom. Figure 4: DFT calculations of electron density. PDOSs for spin-up channel of: ( a ) the Mo atom at the edge and Mo atom within the lattice; ( b ) s , p , and d orbital of Mo-edge atom. ( c ) PDOS of d band of Mo-edge atom, Ag atom from bulk and Ag-slab of 8.32-Å thickness. Electron density on Mo-edge atom is significantly (~11 times) higher than the electron density on Ag atom. Full size image Next, we resolved the PDOS of the Mo-edge atoms into s- , p- and d -orbital electron contributions ( Fig. 4b ). The obtained data indicate that near E f , the PDOS is dominated by d -orbital (Mo) electron states, which are known to actively participate in catalysed reactions [35] . The Mo d electrons form metallic edge states [37] ( Supplementary Note 2 ), which can freely supply electrons to the reactants attached at the edges. To assess how the Mo-edge states are affected by the presence of additional MoS 2 layers, we performed the same analysis for a double-layer MoS 2 strip. Our calculations showed that an interlayer coupling further increases the d -electron PDOS near E f ( Supplementary Note 2 and Supplementary Fig. 9a–d ). In the presence of an external bias, all these d -electron states near E f can be accessed in the reaction, supporting the large observed MoS 2 activity. Finally, we compared our d -orbital PDOS in Mo-edge atoms with that in Ag atoms in two structures: a bulk Ag and a two-dimensional slab Ag (both fcc lattice with a lattice constant of 4.09 Å) of a 8.32-Å thickness (after relaxation) ( Fig. 4c ). We found that the d -band centre for Mo-edge atoms is closer to the Fermi energy level than that in both Ag structures. This can partly explain the high catalytic activity of MoS 2 , since the higher the d -band centre is, the more reactive the metal is due to a lower transition state energy [35] . Moreover, the PDOS of Mo-edge atoms near E f is approximately one order of magnitude higher than the PDOS of Ag atoms, suggesting the availability of the excess of d electrons on the Mo-edge atoms. We believe that both these factors are mainly responsible for the high CO 2 reduction current density of MoS 2 . To reveal the role of EMIM ions in carrying CO 2 molecules, we have also performed quantum molecular dynamics simulations (TeraChem) of the [EMIM–CO 2 ] + complex hydrated in quantum water. We have tested the effect of different pH of the solution on the [EMIM–CO 2 ] + complex stability in several possible configurations. Our simulations reveal that CO 2 most likely binds to EMIM + through the C4/5 protons than through the C2 proton (known to provide stronger binding in vacuum). In this configuration, the complex appears more stable (bond length) and it also provides a better protection against the conversion of CO 2 into HCO 3 − and CO 3 2− species. Our simulations revealed that the EMIM + cation forms a complex [EMIM–CO 2 ] + with CO 2 stabilized by H 2 bonding ( Supplementary Note 3 and Supplementary Fig. 10 ). However, the complex form depends on the pH of the electrolyte. In neutral solution, within ~2 ps, the [EMIM–CO 2 ] + complex reacts with water molecule, forming either the [EMIM–HCO 3 ] or [EMIM–CO 3 ] − complexes ( Supplementary Fig. 10a ). It is well known [38] that in neutral and basic conditions, HCO 3 − and CO 3 2− are the dominant species, respectively. However, our quantum molecular dynamics simulations reveal that in acidic environment, similar to our experimental conditions (pH<4), the [EMIM–CO 2 ] + complex remains stable ( Supplementary Fig. 10 ). These results agree with our previous in situ EMIM–CO 2 complex formation studies [8] . The [EMIM–CO 2 ] + complexes could potentially physisorb (Coulombic and van der Waals coupling) [7] , [8] , [9] at the (negatively charged) MoS 2 cathode, resulting in a close encounter of the CO 2 molecules with the MoS 2 surface. The presence of EMIM + cations around CO 2 molecules can reduce the reaction barrier for electrons passing into CO 2 . Thus, the observed high-CO 2 reduction reaction is attributed to a synergistic action of the MoS 2 catalyst and the EMIM-BF 4 ionic liquid. While EMIM-BF 4 has a crucial role by reducing the overpotential for the reaction, the CO 2 reduction rate is mainly governed by the intrinsic properties of the MoS 2 catalyst. In addition, we measured the work function of MoS 2 through the use of ultraviolet photoelectron spectroscopy. The obtained results indicate that the work function of MoS 2 (3.9 eV) is significantly lower than that of the bulk Ag (4.37 eV) and Ag NPs (4.38 eV) [9] . Due to the low work function of MoS 2 , the abundant metallic-like d electrons in its edge states can take part in the reactions, ultimately resulting in the superior CO 2 reduction performance compared with Ag. Now that we understand that the MoS 2 edges are responsible for the high CO 2 reduction reaction rate, we have synthesized a vertically aligned MoS 2 nanosheet [39] , and observed another factor of two improvements on the CO 2 reduction performance. In brief, a 5-nm thick layer of Mo was deposited on glassy carbon substrate by electron beam evaporation, followed by sulphurization by exposing the film to a sulphur vapour stream at 700 °C. 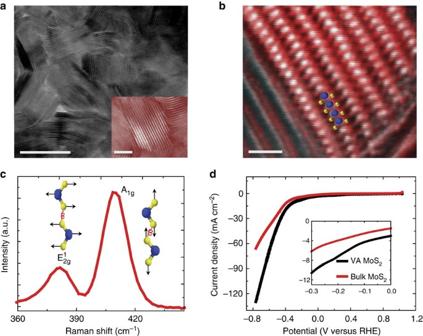Figure 5: Vertically aligned MoS2nanoflakes. (a) Annular bright-field (ABF) STEM images of vertically aligned MoS2(scale bar, 20 nm). STEM analysis (inset) shows the vertically aligned texture of MoS2nanoflakes (scale bar, 5 nm). (b) RGB added image of (G+B) high-angle annular dark-field (HAADF) (R) inverted ABF STEM images of vertically aligned MoS2. High-resolution HAADF STEM image of vertically aligned MoS2(scale bar, 2 nm). Mo atoms are brighter and larger in size in comparison with sulphur atoms due to high atomic number. (c) Raman spectrum for vertically aligned MoS2. (d) CO2reduction performance of bulk MoS2and vertically aligned MoS2represented by VA MoS2. Figure 5a presents a HAADF and annular bright-field image of the vertically aligned MoS 2 nanosheets. While the MoS 2 layers are generally aligned perpendicular to the substrate surface, only a few select sheets can be found which are aligned parallel to the electron beam to allow for atomic resolution imaging ( Fig. 5b ). This image identifies the clearly separated Mo and S atomic columns, as the Mo atoms are heavier and thus appear brighter. The proposed atomic structure of the Mo and S layers is superimposed on the atomic resolution image in Fig. 5b . While the nature of the terminating atoms in these MoS 2 nanosheets cannot be directly visualized in this orientation, previous results have shown that synthesized MoS 2 nanosheets are generally terminated by Mo atoms due to their low-energy state [24] . The vertically aligned MoS 2 samples were further characterized by Raman spectroscopy ( Fig. 5c ). Two essential peaks are clearly visible at 385 cm −1 (in-plane Mo–S phonon mode— E 1 2g mode) and 408 cm −1 (out-of-plane Mo–S phonon mode— A 1 g mode), respectively [21] , [25] , [39] , [40] . The ratio of out-of-plain A 1 g phonon mode to E 1 2g mode is significantly high (~3), which clearly supports the existence of vertically orientated nature of MoS 2 flakes [39] . Figure 5: Vertically aligned MoS 2 nanoflakes. ( a ) Annular bright-field (ABF) STEM images of vertically aligned MoS 2 (scale bar, 20 nm). STEM analysis (inset) shows the vertically aligned texture of MoS 2 nanoflakes (scale bar, 5 nm). ( b ) RGB added image of (G+B) high-angle annular dark-field (HAADF) (R) inverted ABF STEM images of vertically aligned MoS 2 . High-resolution HAADF STEM image of vertically aligned MoS 2 (scale bar, 2 nm). Mo atoms are brighter and larger in size in comparison with sulphur atoms due to high atomic number. ( c ) Raman spectrum for vertically aligned MoS 2 . ( d ) CO 2 reduction performance of bulk MoS 2 and vertically aligned MoS 2 represented by VA MoS 2 . Full size image Figure 5d shows the CO 2 reduction performance of the vertically aligned MoS 2 obtained in similar experimental conditions (that is, 96 mol% water and 4 mol% EMIM-BF 4 ). As expected, CO 2 reduction reaction initiated at low overpotential (54 mV) similar to bulk MoS 2 . Additionally, further improvement has been observed within complete applied potential range ( Fig. 5d ). In the low-applied potential region, vertically aligned MoS 2 exhibits two times higher CO 2 reduction current density compared with the bulk MoS 2 as shown in inset of Fig. 5d . This trend remains also valid in the high-potential region. At −0.764 V, a remarkably high CO 2 reduction current density (130 mA cm −2 ) was recorded for vertically aligned MoS 2 . The high catalytic performance of vertically aligned MoS 2 is attributed to the high density of active sites preferably Mo atoms available for the CO 2 reduction reaction. However, further efforts are needed to understand the nature of edge atoms in the vertically aligned MoS 2 responsible for CO 2 reduction performance. In summary, we have discovered that bulk MoS 2 —a non-precious catalyst and the most versatile member of TMDCs—exhibits the highest observed catalytic performance for the CO 2 reduction. The significantly higher CO 2 reduction current density (relative to noble metal catalysts) is mainly attributed to a high density of d electrons in Mo-terminated edges and also to its low work function. We propose that TMDCs can successfully replace expensive noble metal electrodes, with the promise of higher CO 2 conversion rates and selectivity and can be the most attractive catalyst for future CO 2 reduction applications. MoS 2 characterization Morphology of MoS 2 was visualized at different scales. Optical characterizations were performed by using a Stereo-F ( × 16– × 100 microscope) at × 2 magnification and digital images of bulk MoS 2 (purchased through SPI Supplies) were taken using a 5 mega pixels charge-coupled device camera mounted on the microscope. Scanning electron microscopy was performed to characterize the morphology of the bulk MoS 2 at microscale. The instrument used for characterization is integrated in a Raith e-LiNE plus ultra-high-resolution electron beam lithography system. During imaging, the samples were kept at a distance of 10 mm from the electrons source and the voltage was kept at 10 kV. No particular types of preparation were implemented before imaging. To visualize atomic structure, STEM was performed using a probe-corrected JEOL JEM-ARM200CF equipped with a 200 kV cold-field emission gun. Images were acquired in either the H/LAADF, with the former providing an approximately Z 2 contrast, while the latter is more sensitive to lower angle scattering. A 14 m.r.a.d. probe convergence angle was used for imaging, with the HAADF and LAADF detector angles set to 54–220 and 24–96 m.r.a.d., respectively. Annular bright-field images were also collected to identify S atomic columns, as annular bright-field excels in the imaging of light elements; a collection angle of 7–14 m.r.a.d. was used. For STEM experiments, MoS 2 flakes obtained by mechanical exfoliation of bulk MoS 2 (standard Scotch-tape method) were directly transferred on QUANTIFOIL R 2/1 Holey films with 2-μm circular holes by copper grid (200 mesh, purchased from the Electron Microscopy Sciences). The intensity line profile was attained by using Gatan Digital Micrograph. Both the Web Electron Microscopy Applications Software (WebEMAPS) and CrystalMaker Software programs were also employed to generate and visualize the crystal structures schematically. Raman spectroscopy Raman spectroscopy (Renishaw Raman 2000) was used to detect the MoS 2 in-plane and out-of-plane phonon mode. The spectrum was obtained by exposing small pieces of the samples that is, bulk MoS 2 (without any particular treatment) to 514-nm laser beam (Ar laser, power 10 mW and spot size 10 μm). Ultraviolet photoelectron spectroscopy Surface work function measurements were carried out using ultraviolet photoelectron spectroscopy (UPS). UPS data were acquired with a Physical Electronics PHI 5400 photoelectron spectrometer using He I (21.2 eV) ultraviolet radiation and a pass energy of 8.95 eV. To separate the signal arising from secondary electron emission from the detector to that from the secondary electron emission from the sample, a −9-V bias was applied to the sample using a battery. Electrochemical experiments To examine the catalytic activity of MoS 2 for CO 2 reduction, electrochemical experiments were carried out in a custom made two-compartment three-electrode electrochemical cell ( Supplementary Fig. 3 ). The compartments were separated by a physical barrier using glass frit. Bulk MoS 2 (purchased through SPI Supplies), platinum (Pt) gauze 52 mesh (purchased via Alfa Aesar) and Ag wire (annealed 99.9% metal basis, purchased from Alfa Aesar) were used as working, counter and reference electrode, respectively. EMIM-BF 4 was purchased through Sigma-Aldrich. Electrolytes with different water mole fractions were prepared by adding known volume of deionized water into EMIM-BF 4 . Electrochemical CO 2 reduction experiments were performed in anaerobic CO 2 (AirGas)-saturated electrolyte. The applied voltage was swept between +1.0 and −0.764 V versus RHE with a 15 mV s −1 scan rate. Cyclic voltammetry (CV) curves were then recorded using a Voltalab PGZ100 potentiostat (purchased via Radiometer Analytical SAS) calibrated with a RCB200 resistor capacitor box. The potentiostat was connected to a PC using Volta Master (version 4) software. For chrono-Amperometry measurement, CO 2 concentration was kept constant with bubbling high-purity CO 2 in solution along with mixing during experiment. Current densities were normalized with catalyst geometrical surface area [10] , [16] , [17] , [25] , [26] . Product analysis Electrochemical experimental yields were analysed by GC in SRI 8610C GC system equipped with 72 × 1/8-inch S.S. molecular sieve-packed column and a thermal conductivity detector. Production of CO and H 2 was examined separately. Ultra high-purity helium (purchased through AirGas) was used as a carrier gas for CO detection, whereas ultra high-purity nitrogen (AirGas) was utilized for H 2 detection ( Supplementary Note 4 ). Initially, GC system was calibrated for CO and H 2 . A JEOL GCMate II (JEOL USA, Peabody MA, USA) gas chromatograph/mass spectrometer was further used to prove that yielded CO is only CO 2 electrochemical reduction product. The gas chromatograph was an Agilent 6890Plus (Wilmington DE) equipped with a G1513A auto-injector with 100 vial sample tray connected to a G1512A controller. The GC column was a fused silica capillary column with a nonpolar 5% phenyl 95% dimethylpolysiloxane phase (Agilent HP-5ms Ultra Inert), 30 meters long, 0.25 mm internal diameter, 0.25 μm film thickness. To confirm that the CO product is derived from CO 2 , an isotope 13CO 2 was used as feedstock and GC-Mass spectroscopy was used for gas detection. Mass spectrometer was a bench top magnetic sector operating at a nominal resolving power of 500 using an accelerating voltage of 2,500 v. The spectrometer was operated in full scan EI mode (+ve) with the filament operating at 70 eV scanning from m / z 10 to m / z 400 using a linear magnet scan. The scan speed was 0.2 s per scan. Data analysis was performed using the TSSPro software (Shrader Analytical & Consulting Laboratories, Detroit MI, USA) provided with the spectrometer. Mass calibration was performed using perflourokerosene.The results are discussed in Supplementary Note 5 and Supplementary Fig. 11 . Synthesize of vertically aligned MoS 2 Vertically aligned MoS 2 nanoflakes were grown by chemical vapour deposition using a slightly modified method as reported previously [39] . At first, substrates (glassy carbon) were thoroughly cleaned via rinsing in acetone, methanol and isopropanol solvents sequentially followed by drying in nitrogen flow. Next, a thin layer of Mo (5 nm) was deposited on the substrates by electron beam evaporation (Varian Evaporation System). For sulphurization, Mo-deposited substrates were loaded in the centre of a three-zone furnace (MTI model OTF-1200X) consisting precise temperature and gas flow controller units. The sulphur precursor purchased from Sigma-Aldrich was placed in the upstream of the growing chamber where the maximum temperature reached to 200 °C, above than the sulphur melting point. Before heating process, the chamber was evacuated to 5 mTorr and then the argon (Ar) gas was purged through the chamber to force undesired gases out. Then, the centre of the furnace was heated to 600 °C in 30 min and kept constant for next 15 min. During this growth process, Ar gas was continuously flown (200 SCCM) as a carrier gas. Finally, growth chamber was cooled down to ambient temperature under the protection of Ar gas flow and samples were taken out for further experiments. Physical and electrochemical characteristics of vertically aligned MoS 2 were characterized as previously discussed. Density functional theory calculation We have performed spin-polarized DFT calculations of MoS 2 using SIESTA 3.1 (ref. 41 ) with the Perdew–Burke–Ernzerh of exchange-correlation functional [42] and the norm-conserving Troullier–Martins pseudopotentials [43] to describe valence electrons. The calculations were performed on a real-space grid with a mesh cutoff of 400 Ry within the eigenvalue tolerance of 10 −4 eV, using a DZP (double-zeta basis and polarization orbitals) basis set. The Brillouin zones of the unit cells were sampled by the Monkhorst-Pack grid with a spacing between k-points of Δ k <0.01 Å −1 . The geometry optimization was carried out within the conjugated gradient algorithm, until all the forces are F <0.04 eV per Å and the stress in the periodic direction is σ <0.01 GPa. Quantum molecular dynamics simulations were performed using TeraChem [44] . The energies and forces were evaluated using the B3LYP exchange-correlation functional with 3–21 g basis set with DFT-D dispersion corrections [45] , [46] . The charges were calculated within the Mulliken scheme. How to cite this article: Asadi, M. et al. Robust carbon dioxide reduction on molybdenum disulphide edges. Nat. Commun. 5:4470 doi: 10.1038/ncomms5470 (2014).